Asian pollution climatically modulates mid-latitude cyclones following hierarchical modelling and observational analysis Increasing levels of anthropogenic aerosols in Asia have raised considerable concern regarding its potential impact on the global atmosphere, but the magnitude of the associated climate forcing remains to be quantified. Here, using a novel hierarchical modelling approach and observational analysis, we demonstrate modulated mid-latitude cyclones by Asian pollution over the past three decades. Regional and seasonal simulations using a cloud-resolving model show that Asian pollution invigorates winter cyclones over the northwest Pacific, increasing precipitation by 7% and net cloud radiative forcing by 1.0 W m −2 at the top of the atmosphere and by 1.7 W m −2 at the Earth’s surface. A global climate model incorporating the diabatic heating anomalies from Asian pollution produces a 9% enhanced transient eddy meridional heat flux and reconciles a decadal variation of mid-latitude cyclones derived from the Reanalysis data. Our results unambiguously reveal a large impact of the Asian pollutant outflows on the global general circulation and climate. Air quality has deteriorated in many Asian countries because of their rapid economic development [1] , [2] . For example, as the world’s second largest economy, China has experienced severe air pollution [2] with aerosols or fine particulate matter <2.5 μm (PM 2.5 ) reaching unprecedented high levels across many cities in recent winters. In addition to the impacts of aerosols on air chemistry, visibility, human health and weather [3] , [4] , [5] , intense Asian continental aerosol outflows have been documented from atmospheric field measurements and satellite observations ( Supplementary Fig. 1 ) [1] , [6] , [7] , raising the issue of their potential climate impact. In particular, it has been estimated that about 18 Tg yr −1 of anthropogenic aerosols are exported from East Asia to the Pacific region [7] . Atmospheric aerosols exert a major impact on climate, directly by interfering with the solar radiative transfer and indirectly by influencing cloud formation [8] , [9] . By serving as cloud condensation nuclei, aerosols modify macro- and micro-cloud properties [10] , [11] , [12] and regulate cloud lifetimes and the precipitation efficiency [13] , [14] , [15] , [16] , [17] , [18] . Presently, the estimates of the cloud adjustment by aerosols range from −0.06 to −1.33 W m −2 in the radiative forcing budget, representing the largest uncertainty in climate projections [8] . Also, while atmospheric measurement and modelling studies have revealed invigorated convective cloud systems resulting from elevated aerosol levels [1] , [13] , [16] , the available evidence of the aerosol invigoration effect on clouds is highly variable [8] , [14] , [18] . Much of the uncertainty in the assessment of the aerosol radiative forcing arises from the difficulty to resolve the cloud-scale processes in current global climate models (GCM) [8] . GCM simulations typically predict the response of the climate system under different atmospheric forcing scenarios, but unrealistically represent the microphysical processes of convective clouds. On the other hand, regional cloud-resolving simulations with explicit cloud microphysical and aerosol representations adequately resolve the physical processes of the aerosol–cloud interaction [10] , [11] , but provide little feedback to the large-scale circulation. Previous studies have suggested that the amount of winter deep convective clouds and precipitation have noticeably increased over the north Pacific in recent decades, likely as a result of an increasing Asian pollution outflow [1] , [19] . The wintertime prevalence of mid-latitude cyclones in the Pacific is characterized by the climatological storm track [20] , [21] , and the intensity of the storm track is regulated by several dynamical features of the ocean and atmosphere, including the baroclinicity and upstream seeding of baroclinic eddies [20] , [22] . In addition, the interaction between anthropogenic aerosols and convective clouds may alter the diabatic heating profiles by exerting a radiative forcing on the atmosphere and modifying latent heat from cloud microphysical processes during cyclone development [1] . Here we focus on winter cyclones over the northwest Pacific, directly downstream of the Asian pollution outflow. A hierarchical modelling method is developed by computing the aerosol-induced diabatic forcing from regional and seasonal simulations using a cloud-resolving Weather Research Forecast (CR-WRF) model with explicit bulk microphysics [11] and subsequently incorporating the predicted diabatic heating anomalies into a GCM to assess the climatic impact of Asian pollution. In addition, the National Centers for Environmental Prediction and Department of Energy (NCEP/DOE) Reanalysis data are utilized to assess the inter-decadal variations of the cyclone activity over the northwest Pacific. To quantify the aerosol effects on cloud properties, precipitation, radiation budget and diabatic heating rates and to mimic the Asian pollution outflows, 2-month CR-WRF simulations over the northwest Pacific region are performed under two different aerosol scenarios, that is, a clean maritime case (M-case) and a polluted case with transported aerosols from Asia (P-case). The M-case contains mainly sea salt aerosols to reflect the pristine maritime conditions, while the P-case is dominated by sulphate aerosols. Both cases are initialized on the basis of the results from a global chemical transport model and in-situ atmospheric observations. Our newly developed hierarchical modelling approach resolves the mismatch between simulations by regional mesoscale models and GCMs, allowing a more precise assessment of the global impacts of the cloud-scale processes induced by anthropogenic aerosols. The results from the hierarchical modelling and observational analysis demonstrate that Asian pollution has exerted profound climatic impacts on mid-latitude cyclones over the past three decades. Hierarchical modelling To evaluate the performance of the regional and seasonal simulations by the CR-WRF model, satellite cloud observations from the Moderate Resolution Imaging Spectroradiometer daily data are employed to validate the modelled cyclone development. The simulated cloud properties are consistent with the satellite observation and the CR-WRF model well reproduces the cyclone development over the Pacific ( Fig. 1 ). Additional comparisons of the seasonal cloud fraction and precipitation over the northwest Pacific also exhibit good agreements between CR-WRF simulations and satellite measurements. 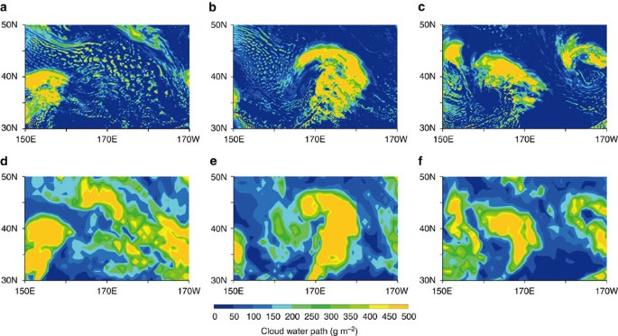Figure 1: Comparison of CR-WRF simulated and satellite-measured cyclone development. CR-WRF simulated cloud water path on 20 (a), 21 (b) and 22 (c) January 2003 and Moderate Resolution Imaging Spectroradiometer (MODIS) Terra Level 3 Daily cloud water path on 20 (d), 21 (e) and 22 (f) January 2003. The differences in the cloud structure away from the storm centre between the observation and model simulation may be partially attributed to the horizontal resolution and microphysics adopted in our CR-WRF. Figure 1: Comparison of CR-WRF simulated and satellite-measured cyclone development. CR-WRF simulated cloud water path on 20 ( a ), 21 ( b ) and 22 ( c ) January 2003 and Moderate Resolution Imaging Spectroradiometer (MODIS) Terra Level 3 Daily cloud water path on 20 ( d ), 21 ( e ) and 22 ( f ) January 2003. The differences in the cloud structure away from the storm centre between the observation and model simulation may be partially attributed to the horizontal resolution and microphysics adopted in our CR-WRF. Full size image Under typical pristine maritime conditions, aerosol concentrations are low, leading to low cloud droplet number concentrations ( Fig. 2a ) and shallow clouds with mainly warm precipitation. As a result, there generally exists a sharp contrast in the lightning distribution between land and ocean [23] , [24] , [25] . Hence, the maritime conditions are highly sensitive to the aerosol perturbation, as previously suggested by in-situ and satellite measurements [26] , [27] . Under the influence of intense aerosol outflows from Asia (P-case), most cloud microphysical properties are significantly altered over the northwest Pacific. For example, the average cloud droplet number concentration is increased by four times because of efficient cloud condensation nuclei activation, but the cloud effective radius is reduced by 40%. Consequently, the conversion from cloud droplets to rain drops is suppressed and warm precipitation of low-level maritime clouds is inhibited. The prolonged water vapour condensation leads to an increase of the cloud liquid water path by 43% ( Fig. 2a ). The increase of 12% in the ice water path ( Fig. 2a ) reflects a more efficient mixed phase process. A 7% enhancement in precipitation is predicted over the entire northwest Pacific domain, with a highest increased precipitation (up to 20%) in convective cloud regions concentrated along the Pacific storm track. The enhanced precipitation is likely linked to a more efficient hydrological circulation, with an enhanced vertical moisture flux from the oceanic surface to the atmosphere. Our predicted precipitation enhancement by Asian pollution in the Pacific region is consistent with a decadal increasing trend of winter precipitation previously identified using the data from the global precipitation climatology project [19] , although the subject of the aerosol effect on precipitation is still debatable [14] , [18] . The maximal vertical convection strength is increased by 40%, revealing considerably invigorated mid-latitude cyclones. 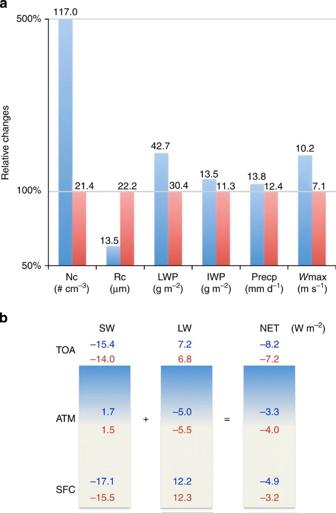Figure 2: Sensitivity of cloud and radiative properties to the aerosol effects. (a) Cloud properties (droplet concentration, Nc; droplet radius, Rc; liquid water path, LWP; ice water path, IWP; precipitation, Precp; maximal updraft velocity at core grids, Wmax) and (b) cloud radiative forcings (shortwave radiation, SW; longwave radiation, LW; net radiation, NET; radiation at the top of the atmosphere, TOA; radiation in the atmosphere, ATM; radiation at the surface, SFC) to the influence of Asian pollution from the CR-WRF simulations. The cloud radiative forcings correspond to the difference between all-sky and clear-sky conditions for the P (blue) and M (red) cases. The aerosol indirect radiative forcing is derived by contrasting the cloud radiative forcing between the clean and polluted conditions. Figure 2: Sensitivity of cloud and radiative properties to the aerosol effects. ( a ) Cloud properties (droplet concentration, Nc; droplet radius, Rc; liquid water path, LWP; ice water path, IWP; precipitation, Precp; maximal updraft velocity at core grids, Wmax) and ( b ) cloud radiative forcings (shortwave radiation, SW; longwave radiation, LW; net radiation, NET; radiation at the top of the atmosphere, TOA; radiation in the atmosphere, ATM; radiation at the surface, SFC) to the influence of Asian pollution from the CR-WRF simulations. The cloud radiative forcings correspond to the difference between all-sky and clear-sky conditions for the P (blue) and M (red) cases. The aerosol indirect radiative forcing is derived by contrasting the cloud radiative forcing between the clean and polluted conditions. Full size image The modified cloud properties by Asian pollution lead to a large variation in the atmospheric radiation flux over the northwest Pacific ( Fig. 2b ). Shortwave cloud radiative forcing at the top of the atmosphere (TOA) and at the surface (SFC) are increased by 1.3 and 1.6 W m −2 ( Fig. 2b ), respectively, both corresponding to about an 11% increase, because of a larger reflectance from brighter clouds. The longwave cloud forcing at TOA is increased by 0.34 W m −2 , because of enhanced high altitude cirrus clouds and widespread anvils that contribute to a warming effect to the radiation budget. Overall, the net cloud radiative forcing is increased by 1.0 W m −2 at TOA and 1.7 W m −2 at SFC over the northwest Pacific because of the influence of Asian pollution. Diabatic heating has been demonstrated to be closely linked to the large-scale dynamics and is determinant in maintaining the baroclinicity of the storm track [28] , [29] . Several components in the CR-WRF simulations contribute to diabatic heating, including shortwave and longwave radiation, latent heat released from the microphysical processes and heating in the planetary boundary layer (PBL) associated turbulent mixing. A comparison of the diabatic heating rates between the two aerosol scenarios ( Fig. 3a ) reveals that there is net heating in the PBL and in the middle troposphere, but net cooling close to the freezing level. The changes in the latent heat release under the different aerosol conditions mainly account for the significant variation in the vertical diabatic heating profile ( Supplementary Fig. 2 ). In the P-case, both latent heating and cooling from the microphysical processes are maximized because of the increased liquid and ice content. The delayed warm rain and enhanced mixed phase processes lead to more efficient latent heat release in the rising air over the warm sectors of the cyclones. Conversely, ice hydrometeors above the freezing level undergo melting and sublimation during settlement, explaining the peak cooling rates at about 850 hPa in the P-case. The exchanges of sensible and latent heats at the air–sea interface and turbulent mixing within the PBL contribute to the large heating rate below 850 hPa ( Fig. 3a ). The spatial distribution of the diabatic heating anomalies by Asian pollution indicates that the modulation of the diabatic heating rates is concentrated over the deep convective region between 30 and 40°N ( Fig. 3b ). 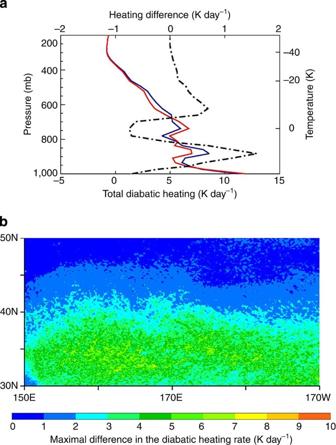Figure 3: Distributions of diabatic heating rates from CR-WRF simulations. (a) Vertical profile of the mean diabatic heating rates. Solid black line denotes the P-case, solid red line denotes the M-case and the dash-dot black line denotes the differences between the two cases (that is, P–M). The upperxaxis corresponds to the difference in the diabatic heating between P and M cases. (b) Spatial distribution of the vertical maximal differences in the diabatic heating rate between the P-case and the M-case (that is, P–M). Figure 3: Distributions of diabatic heating rates from CR-WRF simulations. ( a ) Vertical profile of the mean diabatic heating rates. Solid black line denotes the P-case, solid red line denotes the M-case and the dash-dot black line denotes the differences between the two cases (that is, P–M). The upper x axis corresponds to the difference in the diabatic heating between P and M cases. ( b ) Spatial distribution of the vertical maximal differences in the diabatic heating rate between the P-case and the M-case (that is, P–M). Full size image Simulations with and without the inclusion of the CR-WRF predicted diabatic heating anomalies from Asian pollution are performed using the Community Atmosphere Model version 5 (CAM5). For each diabatic heating scenario, three ensemble runs (that is, with different initial conditions of random perturbations) are carried out to evaluate the statistical variability of the CAM5 simulations. As reflected in the ensemble mean of the high cloud fraction (with altitudes higher than 400 hPa, Supplementary Fig. 3 ), a larger amount of ice clouds occurs in the upper troposphere in the region close to the diabatic heating source (150–180°E). This finding is consistent with a previously identified increasing decadal trend of deep convective clouds from satellite measurements under the influence of Asian pollution [1] . The storm track intensity is quantified by computing the transient eddy meridional heat flux (EMHF) at 850 hPa: where, v ′ and T ′ denote the eddy meridional velocity and eddy temperature departing from the mean seasonal cycles, respectively [30] . The CAM5 simulations reveal that EMHF at 850 hPa is noticeably enhanced under the influence of Asian pollution ( Fig. 4a–c ). As shown in the geographic distribution of the EMHF at 850 hPa ( Fig. 4a,b ), the maxima of the EMHF variances occur at 140E and extend eastward, showing a region of enhanced baroclinic eddy activity. The region with the largest EMHF enhancement of 9.6 K m s −1 occurs at 170°E–170°W and 35–50°N, with an average EMHF enhancement of 1.9 K m s −1 over the entire northwest Pacific. A decreased stability (that is, heating in the middle troposphere and cooling in the upper troposphere) because of the diabatic heating anomalies contributes to a larger baroclinic growth rate [20] and is more favourable for cyclone development [21] . 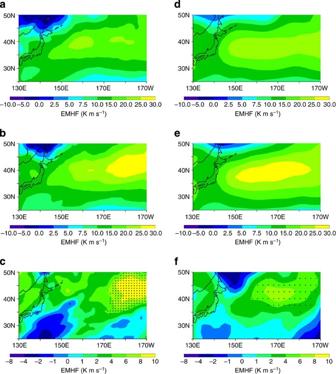Figure 4: Spatial distributions of EMHF at 850 hPa. (a) The ensemble mean of EMHF in the control CAM5 simulation (CTRL), (b) the ensemble mean of EMHF in the CAM5 simulation with the added diabatic forcings from Asian aerosol pollution (AERO) and (c) the difference in EMHF between CTRL and AERO (that is, AERO−CTRL). The EMHF at 850 hPa derived from the NCEP/DOE Reanalysis II data during the decades of (d) 1979–1988 and (e) 2002–2011 and (f) the difference between the two decades (that is (2002–2011)−(1979–1988)) over the northwest Pacific. The dots in (c) and (f) indicate the regions exceeding 99% statistical significance on the basis of Student’st-test. Figure 4: Spatial distributions of EMHF at 850 hPa. ( a ) The ensemble mean of EMHF in the control CAM5 simulation (CTRL), ( b ) the ensemble mean of EMHF in the CAM5 simulation with the added diabatic forcings from Asian aerosol pollution (AERO) and ( c ) the difference in EMHF between CTRL and AERO (that is, AERO−CTRL). The EMHF at 850 hPa derived from the NCEP/DOE Reanalysis II data during the decades of ( d ) 1979–1988 and ( e ) 2002–2011 and ( f ) the difference between the two decades (that is (2002–2011)−(1979–1988)) over the northwest Pacific. The dots in ( c ) and ( f ) indicate the regions exceeding 99% statistical significance on the basis of Student’s t -test. Full size image In our present work the sea surface temperature (SST) is predescribed and, hence, the surface radiation anomalies by aerosols and the associated feedbacks of SST are not accounted for when simulating atmospheric convection and diabatic heating. Our results indicate that the vertical profile of diabatic heating is dominated by the changes in the latent heat release under the different aerosol conditions, with relatively minor contributions from the net cloud radiative forcings. To further evaluate the effect of the surface radiation anomalies by aerosols on SST, additional simulations are performed using the CAM5 coupled with a slab ocean model, showing that SST is insensitive to the net cloud radiative forcing at SFC. The largest difference in the simulated SST with and without the inclusion of the net cloud radiative forcing at SFC and the diabatic heating anomalies induced by Asian pollution is <0.1 K over the northwest Pacific ( Supplementary Fig. 4 ). Observational analysis To corroborate the results of the CAM5 simulations, we evaluate the inter-decadal variations of the Pacific storm track intensity using the NCEP/DOE Reanalysis II data set. The EMHF averaged in January and February over the northwest Pacific (25–50°N, 130°E–170°W) is computed for two 10-year periods, that is, the Reanalysis results from 2002–2011 ( Fig. 4e ) and from 1979–1988 ( Fig. 4d ) to reflect the current (the latest period of the available data) and reference (the earliest period of the satellite era) states of the Asian Pollution outflow, respectively. The earlier reference period (1979–1988) corresponds to the relatively unperturbed maritime conditions from the Asian pollution outflow, preceding the era of major economic developments in Asia [1] , [2] . The comparison of EMHF between the two decadal periods ( Fig. 4f ) reveals a marked difference. The EMHF is considerably enhanced over the northwest Pacific in the latest decade, with an average increase of 1.7 K m s −1 . The region with the largest enhanced EMHF of 7.9 K m s −1 occurs at 160–180°E and 35–45°N. Statistical significance tests indicate that the increased EMHF corresponds to a confidence level of >99%. Furthermore, the analysis of the EMHF from the European Centre for Medium-range Weather Forecasting ERA-Interim Reanalysis data set also supports the increasing trend of the Pacific storm track intensity ( Supplementary Fig. 5 ). The comparison between the CAM5 simulations and Reanalysis shows a similar magnitude and geographic distribution of the EMHF variations under the influence of Asian pollution. The largest EMHF enhancement (that is, by 40% from CAM5 and 30% in Reanalysis) occurs in the region of 150°E–170°W and 35–50°N. Over the entire northwest Pacific, EMHF is increased by an average of 9% for both the CAM5 and Reanalysis results. On the other hand, mid-latitude cyclones are governed by large-scale atmospheric dynamic and thermodynamic conditions, which can also be subject to other anthropogenic forcings, such as global warming induced by greenhouse gases. Our results suggest that the impact of mid-latitude cyclones by Asian pollution is discernable from that caused by other large-scale thermodynamic and dynamic variations. We have strived to develop a novel hierarchical modelling approach by bridging the gap between regional-seasonal cloud-resolving and GCM simulations. Our CR-WRF simulations illustrate invigorated mid-latitude cyclones, with large diabatic heating anomalies induced by Asian pollution over the northwest Pacific. By incorporating the CR-WRF predicted diabatic heating anomalies into the CAM5, we quantify for the first time the climatic modulation of mid-latitude cyclones by Asian pollution and the CAM5 results reconcile the decadal variations of mid-latitude cyclones derived from the Reanalysis data. The remarkable agreement between the CAM5 simulations and Reanalysis results demonstrates unambiguously that Asian Pollution has considerably modified the climatological Pacific storm track over the last three decades. Because of the importance of the Pacific storm track in transporting large amounts of moisture, momentum and sensible heat to higher latitudes and regulating the latitudinal temperature gradient [21] , [31] , we conclude that the global impacts of Asian pollution need to be considered when developing related climate change policies. Regional and seasonal CR-WRF simulations The CR-WRF model with a two-moment bulk microphysical scheme is utilized to assess the impacts of Asian pollution on mid-latitude cyclones over the Pacific [11] . Boundary forcing of the CR-WRF model is derived from the NCEP Final Global Analyses 1° × 1°. The model is configured with two interactive domains ( Supplementary Fig. 6 ). To provide the most coverage of the northwest Pacific, the outer domain has a size of 4,000 × 3,000 km with a 10 km resolution in horizontal and is centred at (40°N and 170°E). The nested inner domain provides a resolution of 2.5 km and covers a 1,000 × 1,500 km area. Real-time global SST analysis data are added into the model as an extra forcing at each input time step. No cumulus cloud parameterization is used. Two-month CR-WRF simulations over the northwest are performed using representative meteorological conditions from 1 January to 28 February 2003. Although the cloud microphysical processes are more explicitly treated using spectral bin microphysics [32] , [33] , such an approach is computationally expensive and rather unrealistic in large-scale and seasonal simulations in the present work. Also, our present work considers only the aerosol indirect forcing. However, the aerosol radiative effect may not be profound over the Pacific region during the wintertime, because of a high cloud frequency and fraction. To investigate the aerosol effect on mid-latitude cyclones, we conducted sensitivity experiments with two aerosol scenarios under identical dynamical and thermodynamical conditions, that is, a polluted case with the consideration of the Asian pollution aerosol outflow (P-case) and a clean maritime case (M-case). Two aerosol species are included in each case: continental aerosols are assumed to mainly contain ammonium sulphate and maritime aerosols are assumed to consist of sodium chloride [34] . Monthly average ammonium sulphate data from the Model of Ozone And Related Tracers Version 2.2 are utilized to interpolate the initial and boundary aerosol fields [35] , [36] . In the P-case, background ammonium sulphate data are initialized using a profile with the maximal number concentration of 2,200 cm −3 at 2.5 km on the basis of aircraft measurements over the northwest Pacific [37] , [38] , [39] , while the initial profile in the M-case has about a maximal ammonium sulphate concentration of 220 cm −3 ( Supplementary Fig. 7 ). The background sea salt is initialized using a profile with the maximal number concentration of 110 cm −3 at the surface for both P-case and C-case. In addition, fixed aerosol profiles derived from the Model of Ozone And Related Tracers are utilized on the domain boundaries to mimic the Asian pollution inflow by advection from the lateral boundary into the model domain under favourable wind conditions. Long-range transport of aerosols to the Pacific storm track region is dominated by anthropogenic sources, while those from natural mineral dust and biogenic aerosols are minimal during the winter season [1] . In this present work, we only consider sulphate aerosols that represent a major constituent in cloud formation [40] , [41] , although secondary organic aerosols, formed from photochemical oxidation of volatile organic compounds [42] , [43] , can also contribute significantly to atmospheric aerosol loading [44] , [45] . Also, there generally is a lack of the long-term record of marine aerosols from in-situ and satellite measurements to infer the unperturbed maritime conditions, while limited satellite observations reveal a trend of increasing aerosol levels during the last three decades over the Pacific [1] . GCM simulations The stand-alone National Centre for Atmospheric Research’s CAM5 is employed in this study and the additional heating computed from CR-WRF is prescribed in the physics package of CAM5 following a previous methodology [46] , [47] . The year 2000 present-day climatological scenario is adopted in the simulations. The SST and sea ice are prescribed in the sensitivity study to exclude the interannual variation of the dynamical factors. The model runs at 0.9° × 1.25° horizontal resolution with 30 vertical levels. Two sets of simulations are designed. The control simulations without the diabatic heating anomalies from Asian pollution (CTRL) are conducted from October to February for each year. The period of the first 3 months is allowed for model spin-up. To evaluate the impacts of the Asian aerosol pollution (AERO), the profiles of the diabatic heating anomalies predicted by the CR-WRF are incorporated to the storm active region over the northwest Pacific (150–180°E and 30–40°N) from January to February. Three winter seasons are simulated with random perturbations on the initial meteorological conditions. The results are averaged over the three winters. There is no assimilation using observational and Reanalysis data within the model domain in our cloud-resolving and global climate simulations. CAM5 is further coupled with a slab ocean model under the frame of NCAR Community Earth System Model to evaluate the effect of the cloud radiative forcing on SST. Simulations for one winter season are conducted with and without the inclusion of the net cloud radiative forcing at SFC and the diabatic heating profile by Asian pollution aerosols calculated from the CR-WRF simulations. Reanalysis data The variation of the Pacific storm track intensity is directly assessed using the NCEP/DOE Reanalysis II. This data set is an improved version of the NCEP/DOE Reanalysis I model. The 6-h meteorological fields at 17 pressure levels are available with a T62 resolution (~210 km) since 1979. The European Centre for Medium-range Weather Forecasting Interim Reanalysis Data is also analysed to validate the results from the NCEP/DOE Reanalysis data. How to cite this article: Wang, Y. et al. Asian pollution climatically modulates mid-latitude cyclones following hierarchical modelling and observational analysis. Nat. Commun. 5:3098 doi: 10.1038/ncomms4098 (2014).